Housing temperature-induced stress drives therapeutic resistance in murine tumour models through β2-adrenergic receptor activation Cancer research relies heavily on murine models for evaluating the anti-tumour efficacy of therapies. Here we show that the sensitivity of several pancreatic tumour models to cytotoxic therapies is significantly increased when mice are housed at a thermoneutral ambient temperature of 30 °C compared with the standard temperature of 22 °C. Further, we find that baseline levels of norepinephrine as well as the levels of several anti-apoptotic molecules are elevated in tumours from mice housed at 22 °C. The sensitivity of tumours to cytotoxic therapies is also enhanced by administering a β-adrenergic receptor antagonist to mice housed at 22 °C. These data demonstrate that standard housing causes a degree of cold stress sufficient to impact the signalling pathways related to tumour-cell survival and affect the outcome of pre-clinical experiments. Furthermore, these data highlight the significant role of host physiological factors in regulating the sensitivity of tumours to therapy. Murine tumour models are used to study nearly all aspects of cancer biology including pre-clinical assessment of novel therapies and identification of novel biomarkers. In fact, the outcomes of mouse studies often dictate the fate of potential cancer therapies and ultimately the implementation and design of clinical trials. As a result, a great deal of effort is being expended to better understand murine models to determine ways to enhance their usefulness as pre-clinical models of disease [1] , [2] , [3] , [4] . Recently, our group has identified a significant factor affecting the outcome of experiments in mice. We found that the standard temperature at which mice are housed impacts basic physiology and tumour progression in experimental mouse models. Specifically, the mildly cool, sub-thermoneutral housing temperature mandated at all research facilities [5] significantly alters both the heat shock protein expression in healthy mice and the anti-tumour immune response [6] , [7] , [8] . In comparison to mice housed at standard temperature (ST; 22 °C), growth of both syngeneic cell lines and carcinogen-induced tumours was significantly delayed in animals housed at thermoneutral temperatures (TT; 30 °C) [8] . Previous studies have shown that mice maintained at ST rapidly lose heat to their surroundings as a result of their large surface area-to-volume ratio [9] requiring increased metabolism to maintain core body temperature at 37 °C (refs 10 , 11 ). Cool temperatures specifically induce the production of a stress hormone, norepinephrine (NE), to activate adaptive thermogenesis [12] . In this context, it is particularly relevant that recent findings have demonstrated that increased levels of NE in both mice and humans can dramatically impact the progression, and especially metastasis, of ovarian, breast and prostate tumours [13] , [14] , [15] , [16] , [17] , [18] , [19] , [20] , [21] . In addition, other studies have revealed that in vitro activation of β-adrenergic receptors can induce tumour-cell proliferation and survival through multiple mechanisms (for example, activation of the MAP Kinase, NFκB and cyclin-dependent kinase pathways) [22] , [23] . Moreover, data has shown that adrenergic signalling promotes the growth of tumour vasculature through production of VEGF and other angiogenic factors [24] , [25] and can impact response to anti-angiogenic therapies. Several recent epidemiological studies have attempted to identify correlations between stress and clinical outcome in cancer patients, and while some of these studies suggest that patients taking β-blockers, competitive antagonists for β-adrenergic receptors, for hypertension or anxiety had improved relapse-free survival in several cancers including breast, ovarian and non-small cell lung cancers [26] , [27] , [28] , [29] , [30] , other studies have failed to identify benefits [31] , [32] , [33] . Based on our previous findings that housing temperature could exert profound effects on tumour growth mediated indirectly through changes in the anti-tumour immune response, we wondered whether chronic, systemic cold stress could also be directly affecting the survival potential of tumour cells. To address this question, we investigated the response of several models of pancreatic cancer to therapies which induce apoptosis. We selected different, clinically relevant therapies that induce apoptosis through the two pathways. Apo2L/TRAIL, a tumour necrosis factor family member, targets cell surface death receptors and activates the extrinsic pathway [34] , [35] , while cisplatin, nab -paclitaxel and erlotinib induce apoptosis [36] , [37] , [38] through the intrinsic pathway. In addition, we explored whether increased signalling through β-adrenergic receptors by NE, which is produced as a normal physiological stress response to cool temperatures, was responsible for the changes in therapeutic efficacy. We report that housing tumour-bearing mice at TTs resulted in a significantly improved baseline response to treatment compared with mice housed at standard room temperatures. Furthermore, we determined that signalling through the β 2 -adrenergic receptors ( ADRB2 ), in response to cold stress-induced NE, resulted in changes to the apoptotic pathway regulation leading to decreases in therapeutic response. Therapies induce greater apoptosis at TT than at ST Based on our previous studies demonstrating that tumour growth was significantly inhibited in mice maintained at TT (30 °C) compared with tumour growth in mice at ST (22 °C), we first sought to determine if the response of tumours to therapies was improved by housing at TT. For these studies, we specifically selected models of pancreatic cancer, as this form of cancer has been previously shown to be responsive to, and possibly even induced by, stress hormones [39] , [40] . We first injected murine Pan02 tumours s.c. into the abdomen of immunocompetent C57BL/6 mice maintained at ST (22 °C). Once tumours reached ~50 mm 3 , mice were randomized and then placed in incubators set at ST or TT (30 °C). After 3 days at ST or TT, mice were treated i.p. with cisplatin (5 mg kg −1 ) twice weekly and tumour growth was monitored. As we saw previously, untreated Pan02 tumours grew more slowly in immunocompetent mice at TT than at ST, and we have previously attributed this to activation of the immune response [8] . In addition, we saw that while cisplatin had only a modest anti-tumour effect at ST, it significantly inhibited tumour growth in mice at TT ( Fig. 1a ), suggesting an increased sensitivity of tumours to cisplatin. 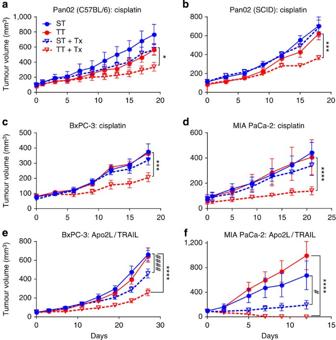Figure 1: Housing mice at TT increases the sensitivity of implantable cell line-derived tumours to therapies. (a) immunocompetent C57BL/6 mice and (b) immunodeficient SCID mice implanted with Pan02 cells in the flank and treated with cisplatin 3 × per week or 2 × per week, respectively. BxPC-3 human pancreatic cancer cell line xenografts in SCID mice treated with (c) cisplatin or (e) Apo2L/TRAIL. MIA PaCa-2 cell line xenografts treated with (d) cisplatin or (f) Apo2L/TRAIL. All data are presented as mean±s.e.m. Statistics by two-way analysis of variance and Tukey analysis: TT control versus TT+Treatment—*P<0.05, ***P<0.001, ****P<0.0001; ST control versus ST+Treatment—#P<0.05,####P<0.0001.N=5–8 per group. Figure 1: Housing mice at TT increases the sensitivity of implantable cell line-derived tumours to therapies. ( a ) immunocompetent C57BL/6 mice and ( b ) immunodeficient SCID mice implanted with Pan02 cells in the flank and treated with cisplatin 3 × per week or 2 × per week, respectively. BxPC-3 human pancreatic cancer cell line xenografts in SCID mice treated with ( c ) cisplatin or ( e ) Apo2L/TRAIL. MIA PaCa-2 cell line xenografts treated with ( d ) cisplatin or ( f ) Apo2L/TRAIL. All data are presented as mean±s.e.m. Statistics by two-way analysis of variance and Tukey analysis: TT control versus TT+Treatment—* P <0.05, *** P <0.001, **** P <0.0001; ST control versus ST+Treatment— # P <0.05, #### P <0.0001. N =5–8 per group. Full size image To specifically explore the potential role of housing temperature in tumour response to therapy, we decided to study the therapeutic response in an immunocompromised model in the absence of the adaptive immune response. Confirming our previous findings, the housing temperature had little effect on the growth of tumours implanted into immunocompromised severe combined immunodeficient (SCID) mice due to the absence of the adaptive immune response [41] , [42] . However, while tumours in SCID mice at ST were unresponsive to cisplatin, tumours in mice at TT were significantly inhibited by cisplatin ( Fig. 1b ). To determine whether this effect of cold stress extended to human tumours, we next assessed the effects of cisplatin on human pancreatic cancer cell line xenografts, MIA PaCa-2 and BxPC-3. In line with our findings in Pan02, these human cell line tumours were also more sensitive to cisplatin when mice were treated at TT compared with those treated at the ST ( Fig. 1c,d ; Supplementary Fig. 1a,b ). In addition, we investigated the response of the cell line xenografts to a second therapy, recombinant human Apo2L/TRAIL, which induces cell death through binding of death receptors and activation of the extrinsic apoptotic pathway [35] , [43] , [44] . These two tumours at TT were also significantly more sensitive to Apo2L/TRAIL compared with tumours in mice at ST, demonstrating that the impact of cold stress on therapeutic response is not limited to cisplatin ( Fig. 1e,f ). We next repeated these experiments using two patient-derived tumour xenografts (PDX): 12424, which we previously characterized as expressing elevated levels of BCL-X L and being highly resistant to Apo2L/TRAIL [45] , and 17624, a moderately Apo2L/TRAIL sensitive tumour. We found that the sensitivity of the patient tumours to Apo2L/TRAIL ( Fig. 2a ), cisplatin ( Fig. 2b ) and nab -paclitaxel ( Fig. 2c,d ; Supplementary Fig. 2a,b ) was enhanced when mice were housed at TT. Cleaved CASP-3 staining revealed that the degree of apoptosis induced by nab -paclitaxel was greater at TT than at ST ( Supplementary Fig. 2c ). Furthermore, the response of a patient lung tumour xenograft to erlotinib, a tyrosine kinase inhibitor which induces apoptosis in cancer cells [36] , was also significantly improved when mice were housed at TT compared with ST ( Supplementary Fig. 2d ). The improved response in the patient-derived lung tumour xenograft shows that this effect is not limited to pancreatic tumours. It is important to note that, confirming our previous findings [8] , mice housed at either ST or TT maintain a normal body temperature ( Supplementary Fig. 3a,b ). This is also true for mice receiving cisplatin treatment ( Supplementary Fig. 3c ). 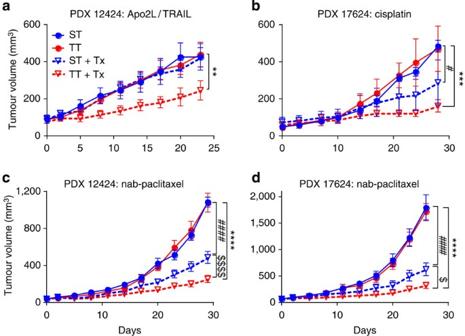Figure 2: Housing mice at TT enhances the response of patient-derived xenografts to therapies. (a) PDX 12424 tumour-bearing mice were treated with Apo2L/TRAIL. (b) PDX 17624 tumour-bearing mice were treated with cisplatin. (c) PDX 12424 and (d) PDX 17624 tumour-bearing mice were treated withnab-paclitaxel. All data are presented as mean±s.e.m. Statistics by two-way analysis of variance and Tukey analysis: TT control versus TT+Treatment—**P<0.01, ***P<0.001, ****P<0.0001; ST control versus ST+Treatment—#P<0.05,####P<0.0001; TT+Treatment versus ST+Treatment–$P<0.05,
    
P<0.0001.N=5 per group. Figure 2: Housing mice at TT enhances the response of patient-derived xenografts to therapies. ( a ) PDX 12424 tumour-bearing mice were treated with Apo2L/TRAIL. ( b ) PDX 17624 tumour-bearing mice were treated with cisplatin. ( c ) PDX 12424 and ( d ) PDX 17624 tumour-bearing mice were treated with nab -paclitaxel. All data are presented as mean±s.e.m. Statistics by two-way analysis of variance and Tukey analysis: TT control versus TT+Treatment—** P <0.01, *** P <0.001, **** P <0.0001; ST control versus ST+Treatment— # P <0.05, #### P <0.0001; TT+Treatment versus ST+Treatment– $ P <0.05, 
    
 P <0.0001. N =5 per group. Full size image To determine if the impact of housing temperature on therapeutic responses, which we observed in tumours implanted s.c., also occurred when tumours were implanted orthotopically, we repeated the experiment in an orthotopic model. In two separate experiments, luciferase expressing MIA PaCa-2 (MIA PaCa-2 luc) cells were implanted into the heads of the pancreas in SCID mice and then treated with either Apo2L/TRAIL or cisplatin. Bioluminescent imaging was performed to monitor tumour growth and recorded as relative flux (photons per s) over the course of the experiment. The results demonstrated that in mice at TT, growth of orthotopic tumours was also inhibited by both therapies, while tumours at ST were resistant ( Supplementary Fig. 4a–d ). Final tumour mass determined at the conclusion of the experiments confirmed that tumours from mice treated at TT were significantly smaller compared with those treated at ST ( Fig. 3a,b ). Taken together, these findings suggest that the sensitivity of the xenografts may be highly plastic and may change in response to different systemic conditions experienced by the host. 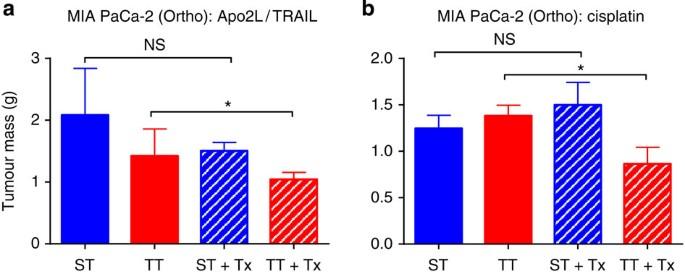Figure 3: The sensitivity of orthotopic pancreatic tumours to therapy is increased in mice at thermoneutrality. MIA PaCa-2 luciferase expressing tumours were implanted orthotopically into the pancreas of SCID mice and treated with: (a) Apo2L/TRAIL or (b) cisplatin. Final mass of recovered tumours was compared at the end of the experiment. All data are presented as mean±s.e.m. Statistics by Student’st-test: *P<0.05; NS, not significant.N=5–6 per group. Figure 3: The sensitivity of orthotopic pancreatic tumours to therapy is increased in mice at thermoneutrality. MIA PaCa-2 luciferase expressing tumours were implanted orthotopically into the pancreas of SCID mice and treated with: ( a ) Apo2L/TRAIL or ( b ) cisplatin. Final mass of recovered tumours was compared at the end of the experiment. All data are presented as mean±s.e.m. Statistics by Student’s t -test: * P <0.05; NS, not significant. N =5–6 per group. Full size image Elevated NE at ST correlates with increased ADRB2 activation Previous work has shown that even moderately cool temperatures can drive the production of a specific catecholamine, NE, which activates body heat production through the process of adaptive thermogenesis [10] , [46] , [47] , [48] . Furthermore, recent reports have demonstrated that NE can act as a pro-survival signal to tumour cells leading to increased metastasis, growth and diminished therapeutic response [49] , [50] , [51] , [52] , [53] , [54] . We hypothesized that mild sub-thermoneutral housing temperatures could elicit a sympathetic cold stress response that would increase levels of NE, which would activate pro-survival pathways in these tumours by binding to β-adrenergic receptors. To investigate this hypothesis, we first confirmed that both β 1 - and β 2 -adrenergic receptors were present on the pancreatic cancer cell lines and patient xenograft cells ( Supplementary Fig. 5a–h ). To confirm that these receptors are not altered directly by treatment, we treated MIA PaCa-2 cells with cisplatin or Apo2/TRAIL in vitro and found that the expression of both β 1 - and β 2 -adrenergic receptors remained unchanged ( Supplementary Fig. 5i,j ). Immunofluorescence for tyrosine hydroxylase demonstrates that NE can be produced locally in the tumour microenvironment ( Supplementary Fig. 6a,b ). Therefore, we next quantitated the NE levels from within the tumours. Interestingly, we found that the intratumoral NE levels of mice at ST compared with those at TT were significantly elevated in BxPC-3 and MIA PaCa-2 and additionally were also trending higher in Pan02 and PDX 12424, ( Fig. 4a–d ). We also assessed plasma levels of NE and found similar elevation in circulating NE levels at ST compared with TT in both naïve and tumour-bearing mice ( Supplementary Fig. 6c–f ). In addition, we investigated the levels of epinephrine (Epi), another catecholamine and corticosterone, a member of another class of stress hormones for which tumour cells express receptors [55] and could therefore affect growth [56] . Analysis of plasma and intratumoral Epi and of faecal corticosterone revealed no significant differences between naïve and tumour-bearing mice at ST and TT conditions ( Supplementary Fig. 7a–i ). 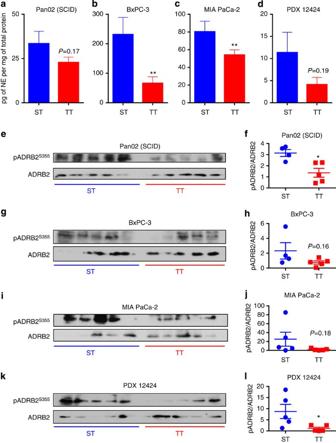Figure 4: Norepinephrine levels and β2-adrenergic receptor activation are increased in the tumours of mice at ST compared with TT. (a–d) Norepinephrine levels were measured in tumour lysates of (a) Pan02 (SCID), (b) BxPC-3, (c) MIA PaCa-2 and (d) PDX 12424 tumour-bearing mice housed at ST and TT. Data is presented as mean±s.e.m. (e–h) Western blot analysis and densitometry quantitation of the ratios of phosphorylated (S355)ADRB2 to ADRB2 and in tumours of (e,f) Pan02 (SCID), (g,h) BxPC-3, (i,j) MIA PaCa-2 and (k,l) PDX 12424 tumour-bearing mice housed at ST and TT. Data ina–dare presented as mean±s.e.m. Statistics by Student’st-test: *P<0.05, **P<0.01.N=5–13 per group. Figure 4: Norepinephrine levels and β 2 -adrenergic receptor activation are increased in the tumours of mice at ST compared with TT. ( a – d ) Norepinephrine levels were measured in tumour lysates of ( a ) Pan02 (SCID), ( b ) BxPC-3, ( c ) MIA PaCa-2 and ( d ) PDX 12424 tumour-bearing mice housed at ST and TT. Data is presented as mean±s.e.m. ( e – h ) Western blot analysis and densitometry quantitation of the ratios of phosphorylated (S355)ADRB2 to ADRB2 and in tumours of ( e , f ) Pan02 (SCID), ( g , h ) BxPC-3, ( i , j ) MIA PaCa-2 and ( k , l ) PDX 12424 tumour-bearing mice housed at ST and TT. Data in a – d are presented as mean±s.e.m. Statistics by Student’s t -test: * P <0.05, ** P <0.01. N =5–13 per group. Full size image To verify that the increased levels of NE within the tumours correlated with increased adrenergic receptor signalling, we quantitated the activation of the more highly expressed β 2 -adrenergic receptor in the tumours of mice maintained at ST and TT by determining the level of phosphorylated receptor as previously described [57] . As expected by the increased NE levels, we found that the phosphorylation of the β 2 -adrenergic receptor at the S355 residue was significantly increased in Pan02 and PDX 12424 tumours of mice housed at ST compared with those at TT and trended towards higher levels in BxPC-3 and MIA PaCa-2 tumours ( Fig. 4e–l ). Cold-stress induces anti-apoptotic changes in tumours in vivo We next investigated possible molecular mechanisms underlying the differences in therapeutic sensitivity of tumours as a result of maintaining the mice at ST and TT conditions. As Apo2L/TRAIL, nab -paclitaxel and cisplatin have well established mechanisms of action involving the extrinsic and intrinsic apoptotic pathways, respectively, we decided to examine the expression of apoptosis regulating proteins that act at the critical juncture of the mitochondria where these two pathways converge. Analysis of the BCL-2 family members, MCL-1, BCL-2 and BCL-X L , revealed that overall levels of these anti-apoptotic molecules were decreased in the tumours of mice maintained at TT compared with ST ( Fig. 5a–j ). Similar changes were observed in MIA PaCa-2 in the orthotopic setting ( Fig. 5k,l ). In addition, we analyzed levels of FLIP L, an inhibitory molecule upstream of the mitochondria, but found no difference in the expression between ST and TT ( Supplementary Fig. 8 ). Overall, these findings indicate that the stress induced by housing temperature increases the expression of anti-apoptotic signalling molecules in tumours, although the specific pattern varies depending on the tumour. 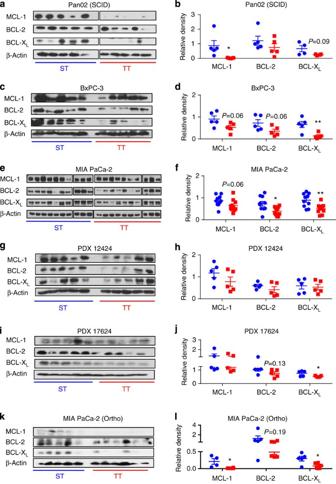Figure 5: Expression of anti-apoptotic molecules is decreased in untreated tumours from mice at TT versus ST. Western blot analysis and densitometry (protein of interest/β-Actin) of MCL-1, BCL-2 and BCL-XLfrom (a,b) Pan02 (SCID), (c,d) BxPC-3, (e,f) MIA PaCa-2, (g,h) PDX 12424, (i,j) PDX 17624 and (k,l) orthotopic MIA PaCa-2 tumours of mice housed at ST and TT. Statistics by Student’st-test: *P<0.05, **P<0.01.N=5–10 per group. Figure 5: Expression of anti-apoptotic molecules is decreased in untreated tumours from mice at TT versus ST. Western blot analysis and densitometry (protein of interest/β-Actin) of MCL-1, BCL-2 and BCL-X L from ( a , b ) Pan02 (SCID), ( c , d ) BxPC-3, ( e , f ) MIA PaCa-2, ( g , h ) PDX 12424, ( i , j ) PDX 17624 and ( k , l ) orthotopic MIA PaCa-2 tumours of mice housed at ST and TT. Statistics by Student’s t -test: * P <0.05, ** P <0.01. N =5–10 per group. Full size image Previous works by others have described the effects of NE on tumour cells in vitro and in vivo. These reports demonstrated that activation of the adrenergic receptors by stress hormones such as NE can initiate multiple downstream events including the phosphorylation of both the transcription factor CREB, which can drive the expression of numerous genes that govern proliferation and survival and the pro-apoptotic protein BAD, which leads to its inactivation [16] , [19] . To further characterize the effects of the cold stress on tumour-bearing mice, we compared the phosphorylation status of CREB S133 and BAD S112 , which are modification sites for these molecules in response to adrenergic receptor signalling sources in tumours of mice housed at ST and at TT. In Pan02, BxPC-3 and PDX 12424, we observed higher levels of phosphorylated CREB S133 ( Fig. 6a–f ). Higher levels of phosphorylated BAD S112 were detected in Pan02, BxPC-3, PDX 12424, PDX 17624 and orthotopic MIA PaCa-2 ( Fig. 6a–j ). 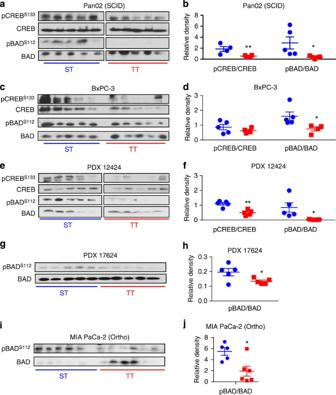Figure 6: Phosphorylation of CREB and BAD in untreated, control tumours is decreased at TT compared with ST. Western blot analysis and densitometry quantitation (phosphorylated protein/unphosphorylated protein) of pCREBS113or pBADS112from (a,b) Pan02 (SCID), (c,d) BxPC-3 and (e,f) PDX 12424 and (g,h) PDX 17624 and (i,j) orthotopic MIA PaCa-2 tumour-bearing SCID mice housed at ST and TT. Statistics by Student’st-test: *P<0.05, **P<0.01.N=5 per group. Figure 6: Phosphorylation of CREB and BAD in untreated, control tumours is decreased at TT compared with ST. Western blot analysis and densitometry quantitation (phosphorylated protein/unphosphorylated protein) of pCREB S113 or pBAD S112 from ( a , b ) Pan02 (SCID), ( c , d ) BxPC-3 and ( e , f ) PDX 12424 and ( g , h ) PDX 17624 and ( i , j ) orthotopic MIA PaCa-2 tumour-bearing SCID mice housed at ST and TT. Statistics by Student’s t -test: * P <0.05, ** P <0.01. N =5 per group. Full size image Adrenergic signalling in vitro induces resistance to therapy The above experiments suggest that tumours at ST respond to elevated levels of NE by increasing expression of anti-apoptotic molecules (BCL-2, BCL-X L and MCL-1) and inactivating the pro-apoptotic molecule BAD. To determine if activation of the β-adrenergic receptors on tumour cells themselves could directly affect these changes, we stimulated cells in vitro with isoproterenol, a non-selective β 1 - and β 2 -adrenergic agonist. After stimulating with either 100 nM or 1 μM for 24 or 48 h, protein expression was assessed. In response to β-adrenergic receptor activation, the expression of BCL-2 family members was increased in a cell line-specific pattern in the different tumour lines; however, phosphorylation of BAD S112 was significantly increased in response to β-adrenergic stimulation in all lines ( Fig. 7a–l ; Supplementary Fig. 9a–c ). Next, to determine if the increased expression of anti-apoptotic molecules induced by β-adrenergic signalling results in increased resistance to therapies, tumour cells were pre-treated with 1 μM of isoproterenol followed by treatment with either Apo2L/TRAIL (1 μg ml −1 ) for 4 h or cisplatin (10 μg ml −1 ) for 24 h and then assessed for induction of apoptosis as determined by cleaved CASP-3 levels. Following β-adrenergic receptor activation, the levels of cleaved CASP-3 in Apo2L/TRAIL-treated cells were significantly less than in untreated cells (BxPC-3, 27.43 to 18.97%; MIA PaCa-2, 53.9 to 27.32%; Fig. 8a–d ) indicating that these cells were protected from apoptosis. 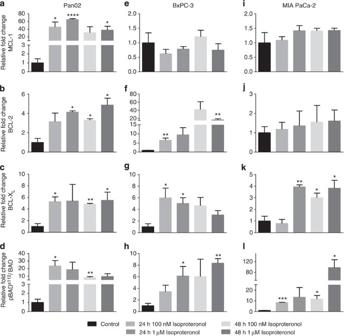Figure 7:In vitroactivation of β-adrenergic receptors increases expression of anti-apoptotic proteins. (a–d) Pan02, (e–h) BxPC-3, (i–l) MIA PaCa-2 tumour cells were treated with 1 or 100 μM of the β-adrenergic receptor agonist, isoproterenol, for 24 or 48 h. Western blot analysis and relative densitometry quantitation for (a,e,i) MCL-1, (b,f,j) BCL-2, (c,g,k) BCL-XLand (d,h,l) relative fold change in the pBADS112to BAD ratio. All data is presented as mean±s.e.m. Statistics by Student’st-test: *P<0.05, **P<0.01, ***P<0.001, ****P<0.0001. Experiments were performed in triplicate. Figure 7: In vitro activation of β-adrenergic receptors increases expression of anti-apoptotic proteins. ( a – d ) Pan02, ( e – h ) BxPC-3, ( i – l ) MIA PaCa-2 tumour cells were treated with 1 or 100 μM of the β-adrenergic receptor agonist, isoproterenol, for 24 or 48 h. Western blot analysis and relative densitometry quantitation for ( a , e , i ) MCL-1, ( b , f , j ) BCL-2, ( c , g , k ) BCL-X L and ( d , h , l ) relative fold change in the pBAD S112 to BAD ratio. All data is presented as mean±s.e.m. Statistics by Student’s t -test: * P <0.05, ** P <0.01, *** P <0.001, **** P <0.0001. Experiments were performed in triplicate. 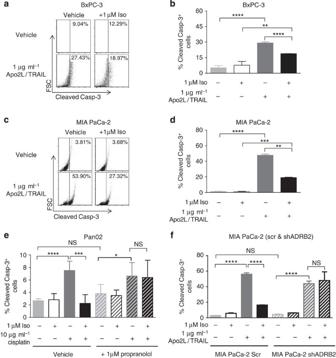Figure 8:In vitroactivation of β-adrenergic receptors on pancreatic tumour-cell lines increases resistance to Apo2L/TRAIL. (a,b) BxPC-3 and (c,d) MIA PaCa-2 tumour cells were incubated with 1 μM isoproterenol for 48 h and then treated with 1 μg ml−1of Apo2L/TRAIL for 4 h. Cell death is evaluated by flow cytometry of cleaved CASP-3-positive cells. (e) Pan02 cells were incubated with 1 μM isoproterenol for 48 h and then treated with 10 μg ml−1of cisplatin for 4 h in the presence (hatched bars) or absence (solid bars) of 1 μM propranolol. (f) MIA PaCa-2 shADRB2 cells (hatched bars) or scramble (solid bars) were treated with 1 μM isoproterenol for 48 h and then 1 μg ml−1of Apo2L/TRAIL for 4 h. Data inb,d–fare presented as mean±s.e.m. Statistics by Studentt-test: NS, not significant, *P<0.05, **P<0.01, ***P<0.001, ****P<0.0001. Experiments were performed in triplicate. Full size image Figure 8: In vitro activation of β-adrenergic receptors on pancreatic tumour-cell lines increases resistance to Apo2L/TRAIL. ( a , b ) BxPC-3 and ( c , d ) MIA PaCa-2 tumour cells were incubated with 1 μM isoproterenol for 48 h and then treated with 1 μg ml −1 of Apo2L/TRAIL for 4 h. Cell death is evaluated by flow cytometry of cleaved CASP-3-positive cells. ( e ) Pan02 cells were incubated with 1 μM isoproterenol for 48 h and then treated with 10 μg ml −1 of cisplatin for 4 h in the presence (hatched bars) or absence (solid bars) of 1 μM propranolol. ( f ) MIA PaCa-2 shADRB2 cells (hatched bars) or scramble (solid bars) were treated with 1 μM isoproterenol for 48 h and then 1 μg ml −1 of Apo2L/TRAIL for 4 h. Data in b , d – f are presented as mean±s.e.m. Statistics by Student t -test: NS, not significant, * P <0.05, ** P <0.01, *** P <0.001, **** P <0.0001. Experiments were performed in triplicate. Full size image Moreover, treatment with the β 1 -, β 2 -adrenergic receptor antagonist, propranolol, abrogated the resistance to therapy induced by isoproterenol. The improved response following treatment with propranolol demonstrates a critical role for β-adrenergic receptor signalling in mediating the increased resistance to apoptotic cell death ( Fig. 8e , Supplementary Fig. 11a ). A specific role for the β 2 -adrenergic receptor is revealed by short hairpin RNA knockdown of the β 2 -adrenergic receptor ( Supplementary Fig. 10a,b ), which also abrogates resistance ( Fig. 8f , Supplementary Fig. 11b ). In addition, cell viability was assessed in vitro by MTT assay and was shown to be significantly increased in response to β-adrenergic receptor activation ( Supplementary Fig. 11c–h ). These findings from experiments conducted with tumour cells in vitro , in the absence of other cell types which are found in the tumour microenvironment, indicate that direct activation of β-adrenergic receptors on tumour cells, particularly the β 2 -adrenergic receptor, can protect cancer cells from therapies which induce apoptosis. β-adrenergic blockade reverses in vivo resistance at ST Finally, to explore whether the resistance to therapies induced by cold stress in vivo is also mediated through activation of the β-adrenergic receptors, we next treated tumour-bearing mice with a therapy in combination with propranolol at both ST and TT conditions. We hypothesized that inhibiting the receptor signalling would increase the sensitivity of the mice to therapies at ST; however, since the levels of NE are already lower in the tumours of mice at TT than at ST, we expected to see little benefit in blocking the receptor in these TT animals. As predicted, mice which were housed at ST and treated with a combination of propranolol and Apo2L/TRAIL displayed significantly enhanced responses that were similar to responses of tumours in mice treated with Apo2L/TRAIL under TT alone conditions ( Fig. 9a,b ). Moreover, treatment of the tumours at TT conditions with propranolol in combination with Apo2L/TRAIL did not further improve the response, suggesting that the β-adrenergic receptor blockade is efficacious only in organisms which are under stress. To determine if the change in response was due to direct effects of β 2 -adrenergic signalling on the tumour cells, we tested the response of MIA PaCa-2 shADRB2 cells to treatment with Apo2L/TRAIL at ST and TT conditions. Knockdown of the receptor did not affect tumour growth when mice were housed at ST or TT compared with scrambled controls ( Fig. 9c ). In addition, in mice housed at TT, both scramble control tumours and shADRB2 tumours had responses to single agent treatment. However, when mice were treated with Apo2L/TRAIL, shADRB2 tumours at ST had an improved response compared with scramble control tumours, indicating that the β 2 -adrenergic receptor mediated the resistance observed at ST conditions ( Fig. 9c ). 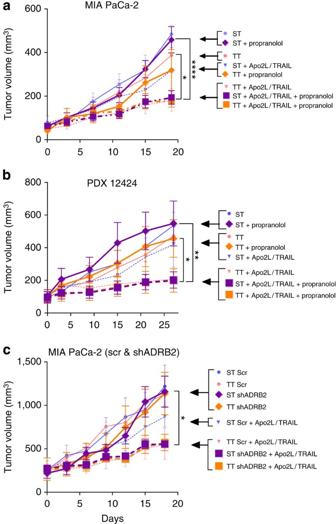Figure 9: Inhibition of β-adrenergic signalling increases tumour response to Apo2L/TRAIL at ST but not at TT. ST and TT mice bearing (a) MIA PaCa-2 and (b) PDX 12424 were treated with Apo2L/TRAIL with or without propranolol. (c), MIA PaCa-2 cells were transfected with shADRB2 and implanted into the abdomen of SCID mice housed at ST and TT. These mice were treated with Apo2L/TRAIL with or without propranolol. All data are presented as mean±s.e.m. Statistics by two-way analysis of variance: *P<0.05, **P<0.01, ****P<0.0001.N=4–6 per group. Figure 9: Inhibition of β-adrenergic signalling increases tumour response to Apo2L/TRAIL at ST but not at TT. ST and TT mice bearing ( a ) MIA PaCa-2 and ( b ) PDX 12424 were treated with Apo2L/TRAIL with or without propranolol. ( c ), MIA PaCa-2 cells were transfected with shADRB2 and implanted into the abdomen of SCID mice housed at ST and TT. These mice were treated with Apo2L/TRAIL with or without propranolol. All data are presented as mean±s.e.m. Statistics by two-way analysis of variance: * P <0.05, ** P <0.01, **** P <0.0001. N =4–6 per group. Full size image To determine if loss of signalling through the β-adrenergic receptors resulted in decreased expression of anti-apoptotic proteins to levels seen in tumours from mice housed at TT alone, we investigated the levels of these proteins by Western blot. As previously observed, MIA PaCa-2 tumours in mice housed at TT had significantly decreased expression of BCL-2 and BCL-X L , as well as decreased levels of pBAD S112 . Treatment of these tumours at TT with propranolol did not further alter the expression of these proteins; however, blockade of β 1 -, and β 2 -adrenergic receptor signalling at ST with propranolol resulted in significant decreases in the expression of BCL-2 and BCL-X L , ( Fig. 10a,c ) and diminished phosphorylation of Bad S112 ( Fig. 10b ). Similar findings were also seen in the PDX 12424, which had decreased levels of pBad S112 in response to propranolol treatment at ST conditions ( Fig. 10d,e ). These findings demonstrate that β-adrenergic receptor signalling in cold-stressed mice can increase the expression of anti-apoptotic molecule expression and alter the efficacy of apoptosis-inducing therapies and this can be reversed by adrenergic receptor blockade. 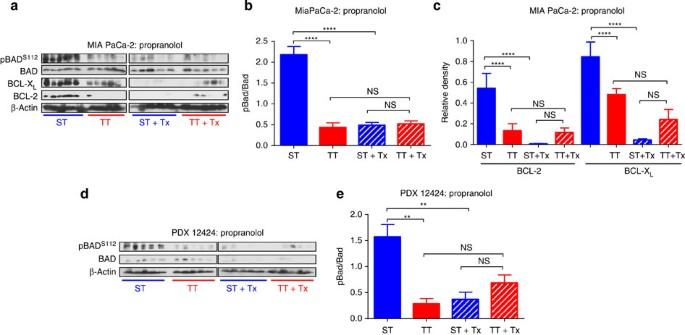Figure 10: Propranolol treatment significantly decreases the expression of anti-apoptotic proteins in tumours from ST mice. Western blot analysis and densitometry of anti-apoptotic molecules from (a–c) MIA PaCa-2 and (d,e) PDX 12424 tumour-bearing mice treated with propranolol. Data inb,c,eare presented as mean±s.e.m. Statistics by Student’st-test: **P<0.01, ****P<0.0001.N=5 per group. Figure 10: Propranolol treatment significantly decreases the expression of anti-apoptotic proteins in tumours from ST mice. Western blot analysis and densitometry of anti-apoptotic molecules from ( a – c ) MIA PaCa-2 and ( d , e ) PDX 12424 tumour-bearing mice treated with propranolol. Data in b , c , e are presented as mean±s.e.m. Statistics by Student’s t -test: ** P <0.01, **** P <0.0001. N =5 per group. Full size image Murine models have become essential tools for evaluation of therapeutic efficacy in cancer research; however, recent work implicates housing conditions, such as lack of exercise, overeating and housing density as underappreciated sources of variability in pre-clinical research studies [58] , [59] . Here we have examined the role of housing temperature, which is another seldom considered variable that can potentially influence experimental outcomes [60] , [61] . Our data reveal that the response of several pancreatic tumour models to cisplatin, Apo2L/TRAIL or nab -paclitaxel can be enhanced merely by housing mice at TT, thereby alleviating cold stress. Since the catecholamine, NE, mediates the physiological response to cold stress, we examined levels of NE at ST and TT and found that increased therapeutic sensitivity correlated with decreased levels of NE in the tumour microenvironment and sensitivity could be increased by administration of a β-adrenergic receptor antagonist at ST. Furthermore, we found that activation of the β 2 -adrenergic receptor, based on the increased phosphorylation at S355, was higher in the tumours of mice at ST than at TT. These results contribute to a growing body of literature, revealing NE as a potent tumour promoting molecule that can drive growth and metastasis [62] . Sastry et al . [16] have shown, in vitro , that Epi can protect prostate and breast cancer cells from apoptosis induced by a PI3K inhibitor through phosphorylation of BAD, while Hassan et al . [19] have revealed a link between stress and prostate tumour progression in vivo leading to BAD phosphorylation which also can protect against apoptosis; in both cases, this protection can be reversed by administration of an ADRB2 antagonist. Others have also demonstrated that stress upregulates expression of certain members of the anti-apoptotic BCL-2 family which can be inhibited by ADRB2 blockade [22] , [63] . In tumours grown in mice at TT, we found decreased expression of several critical intratumoral anti-apoptotic molecules which could explain the increased sensitivity to the apoptosis-inducing cytotoxic therapies investigated here. In addition, we discovered that increased sensitivity to therapy occurring at TT could be replicated by inhibiting adrenergic signalling in ST mice, either by pharmacologic blockade or short hairpin RNA-mediated silencing of ADRB2 . Inhibition of adrenergic signalling at ST also led to decreased expression of anti-apoptotic proteins. These findings reveal that mild stress imposed by cool housing conditions can activate the same anti-apoptotic mechanisms seen in vivo in classic stress experiments or in vitro by β-adrenergic receptor agonists, and show that pre-existing levels of stress should be taken into account when assessing the sensitivity of any given tumour to novel therapies. The differential roles that Epi and NE play in the progression of cancer and protection of tumours from apoptosis still require further exploration. In classic stress experiments, elevation of Epi has been reported in the plasma of mice [19] , but in epidemiological studies, NE levels were found to be elevated in the tumours of patients [20] . Due to the complexities of tumour cells, each type of malignancy may respond differently to various stress hormones. In our models, elevated levels of NE, but not Epi, were found in the tumours of mice at ST compared with TT. The source of this NE remains to be identified, but it is likely that both macrophages [48] and sympathetic nerves [64] contribute to the NE levels in the tumour microenvironment. Overall, our results indicate that the anti-apoptotic, pro-tumour effects of stress induced in classic restraint and social isolation experiments are already activated at ‘baseline’ in tumours of control laboratory mice. Tumours also differ in terms of the specific responses to NE as we saw specific patterns of anti-apoptotic molecules upregulated in different tumours. Also, in our studies, MIA PaCa-2 and BxPC-3 tumours, which had significantly different levels of NE at ST and TT, did not show statistically different levels of receptor phosphorylation. One possibility for the discrepancy may be due to desensitization of the receptor, since both of these tumours had much higher levels of intratumoral NE compared with the other models. Thus, these receptors may have reached their maximum signalling potential, and to prevent cellular damage from overstimulation, have induced a negative feedback system. However, this aspect of β 2 -adrenergic receptor biology needs further exploration. These results are a first step in recognizing how temperature-induced adrenergic signalling affects pre-clinical tumour models, but a fuller understanding of the mechanisms involved is still needed. In particular, our work specifically implicates the β 2 -adrenergic receptor as the main driver for resistance in pancreatic tumours under mild cold stress (standard) conditions, and this correlates with reports that blockade of the β 2 -adrenergic receptor can affect tumour progression in certain cancer types [23] , [65] , [66] . Supporting the role of the β 2 -adrenergic receptor are several epidemiological studies of patients indicating that those on pan-β-blockers have improved survival outcomes compared with patients taking β 1 - specific blocking agents [26] , [27] . However, the differential contributions of the β 1 and β 2 receptors still need further exploration. It would be particularly interesting to carry out gain-of-function experiments in which tumour-bearing mice would be treated with ADBR1- and ADBR2-specific agonists to ascertain the relative role of these two receptors in inducing therapeutic resistance. In the future it will also be important to evaluate the role of ADBR3 signalling in the tumour microenvironment since Magnon et al . [64] have shown that prostate tumour development was more delayed in double knockout mice (ADRB2 −/− and ADRB3 −/− ) than in mice with either individual receptor knocked out. In addition, recent work has identified the presence of β 3 -adrenergic receptors on melanomas [67] . This finding comes as a surprise since the tissue expression of β 3 -adrenergic receptors is much more restricted compared with the β 1 - and β 2 - adrenergic receptors. Specific pharmacologic blockade of the β 3 -adrenergic receptors was able to significantly control tumour growth, suggesting that this receptor isoform may also have an important role in tumour progression and may present another possible drug target [67] . Others have demonstrated a pro-angiogenic role for stress [49] , [50] and while we did not address the effects of ST versus TT on tumour vasculature, this is an important question for future studies since variations in blood flow and/or hypoxia have implications for drug delivery and tumour sensitivity. There are likely other indirect effects of NE signalling in the tumour microenvironment, as well (for example, on immune cells) [62] , [68] . Although, we have not specifically examined the effect of housing temperature on innate immune cells such as neutrophils, macrophages or natural killer cells, it is possible that they could also influence the response of tumours to therapies at different ambient temperatures. In addition, work by Madden et al . [69] have shown that in a model of social isolation, increased NE levels were associated with an accumulation of suppressive immune cells. Nevertheless, the in vitro studies reported here support the conclusion that NE has significant direct effects on tumour cells and their therapeutic resistance. Experiments designed to assess the effects of stress in mouse models are classically conducted by imposing physical (restraint) or psychological (social isolation) stress on ‘control’ mice. From our data, it is clear that these experimental stressors are imposed on animals that are already under physiologically significant cold stress. Moreover, while other groups have established that temperature can alter systemic drug metabolism [70] , and therefore pharmacokinetics in laboratory rodents, our findings reveal another cause for concern. Our work demonstrates that cold stress can also affect therapeutic efficacy by modulating survival pathways within cells. Conversely, unforeseen side-effects may also become more apparent in mice housed at thermoneutrality and this aspect of drug evaluation remains to be investigated. Currently, we are not advocating that housing mice at TT versus current ST is more ‘correct’, or a more accurate representation of human patients. However, it is clear that tumours exhibit a wide spectrum of responses to therapies under different conditions and that this should be taken into consideration in pre-clinical studies. Ultimately, establishing accurate baseline responses is critical for the optimization of treatment strategies and the development of novel drug combinations. Cell culture MIA PaCa-2 and BxPC-3 cell lines were obtained from ATCC. Pan02 was obtained from the NCI Tissue Repository. BxPC-3 and Pan02 cells were cultured in standard RPMI 1640 medium supplemented with 10% foetal calf serum, 1% L -glutamine, 1% penicillin–streptomycin. MIA PaCa-2 was cultured in DMEM enriched with previously mentioned additives and 5% horse serum. Western blot Tumours samples were harvested and immediately snap frozen. Protein was extracted with lysis buffer (containing 0.5 M Tris, 2.5 M NaCl, 500 mM NaF and 10% non-ionic P 40 with the addition of protease inhibitors: 200 mM Na 3 VO 4 , 0.5 M β-glycerophosphate, 0.25 M NaPPi, 0.1 M PMSF, 1 mg ml −1 leupeptine, 0.1 M benzamidine and 1 mg ml −1 aprotinin). Total protein was quantitated by colorometric protein assay (Bio Rad) and read by plate reader (Biotek HT) at 680 nm. Proteins were resolved by SDS–PAGE, transferred to a polyvinylidene difluoride membrane (Millipore) and blocked with 3% BSA (Santa Cruz Biotechnology, sc-16719-R) in Tris buffered saline with tween 20 (TBS-T). Membranes were probed for BCL-X L (2764), Mcl-1 (D35A5), BCL-2 (non-species specific; 2876 and human specific; 2872 antibodies), phospho-Creb S133 (9198), phospho-Bad S112 (Cell Signaling) and phospho-ADRB2 S355 (Santa Cruz; sc-22191-R). Membranes were also probed for Bad (Abcam; ab32445), CREB (ThermoScientific) and FLIP L (AbdSerotec; MCA4262Z). β-actin (Sigma; A5441) was used as a loading control. Anti-rabbit horseradish peroxidase (Enzo Life Sciences; ADI-SAB-300-J) and anti-mouse alkaline phosphatase (AP) (Vector Labs; AP-2000) secondaries were used and developed with ECL-substrate (Bio Rad) or AP Substrate (Bio Rad), respectively, on film (lipopolysaccharide). All primary antibodies were diluted 1:1,000 in TBS-T, β-actin was diluted at 1:10,000 in TBS-T. Secondary anti-rabbit horseradish peroxidase was diluted at 1:3,000 in TBS-T, anti-mouse AP was diluted at 1:10,000 in TBS-T. Images were scanned (Epson Perfection 2450) and densitometries were calculated by ImageJ software. Images have been cropped for presentation. Uncropped images of original Western blots are presented in Supplementary Figs 12–24 . Immunohistochemistry PDX 12424 tumours treated with nab -paclitaxel were FFPE. Heat-mediated antigen retrieval was carried out with DAKO Target Retrieval Solution and sections were stained for cleaved CASP-3 (Cell Signaling; 9661), followed by biotinylated goat anti-rabbit (Jackson Immunoresearch; 711-066-152) and ABC-RTU (Vector Laboratories, Inc, Burlingame CA, USA) and visualized with Impact DAB (Vector). Labelled cells were quantified by counting five random fields/slide at × 400 magnification; tumours from three mice per group were used. Since tumours naturally have large areas of necrosis, counts were made by avoiding these areas. Immunofluorescence Pan02 tumours grown in C57BL/6 mice at ST were recovered and embedded in OCT embedding medium. Frozen sections (8–10 μm) were fixed in cold acetone and stained for tyrosine hydroxylase (Millipore; AB152), followed by biotinylated goat anti-rabbit antibody, ABC-RTU, and visualized with Tyramide Signal Amplification kit for TRITC (Perkin Elmer). Identification of β-adrenergic receptors on tumour cells The expression of cell surface β 1 - and β 2 -adrenergic receptor was done by flow cytometry. In vitro tumour-cell lines were harvested and stained with antibodies against β 1 -adrenergic and β 2 -adrenergic receptors (Santa Cruz Biotechnology; sc-567, sc-81578). Patient tumour xenografts were harvested from SCID mice and dissociated using a Miltenyi gentleMACS Dissociator (Miltenyi) as per the manufacturer’s instructions. Single cells were re-suspended in PBS with 0.1% BSA and stained with antibodies against β 1 - and β 2 -adrenergic receptor. Mouse cells were excluded from analysis using antibodies against H2K d (eBioscience; 13-5998-82). β 1 - and β 2 -adrenergic receptor antibodies were diluted to 1 μl per 10 6 cells, H2K d was diluted to 0.5 μl per 10 6 cells, flow cytometry was performed on an LSR II flow cytometer and data was analyzed using FCS Express software (DE Novo). Protein expression following adrenergic receptor activation About 5 × 10 5 tumour cells were plated in triplicate overnight and then treated with 100 nM or 1 μM isoproterenol HCL in serum-free media for 24 or 48 h. Cells were harvested on ice with protein lysis buffer and Western blots were performed as described above. Cleaved CASPASE-3 activation About 10 5 tumour cells were plated in triplicate overnight and then treated with 1 μM isoproterenol HCL in serum-free media for 48 h. Pan02 cells were pre-treated with 1 μM of propranolol HCL for 30 min prior to the addition of isoproterenol. The cells were then treated with either 1 μg ml −1 of Apo2L/TRAIL (Genentech) for 4 h or 10 μg ml −1 of cisplatin (APP Pharmaceuticals, LLC) for 24 h. Detached and adherent cells were harvested with 0.25% trypsin and washed with PBS. Cells were fixed and permeabilized with BD Cytoperm/Cytofix kit (BD Biosciences) according to manufacturer’s instructions and stained for intracellular flow cytometry with anti-cleaved CASPASE-3 antibody (BD Biosciences; 560627). Analysis of data was performed as previously described. MTT assay About 10 4 cells were plated in quadruplicate in a 96-well plate. Cells were treated in culture with isoproterenol HCL as described above. Afterwards, media was removed and serum-free, phenol red-free media containing increasing concentrations of either cisplatin or Apo2L/TRAIL were added for 48 h or 12 h, respectively. The media was later removed and 100 μl of 1 mg ml −1 MTT assay reagent (Invitrogen) in media was added to the wells and incubated at 37 °C for 3 h. When incubations were completed, the MTT assay reagent was removed and cells were dissolved in MTT Solvent (4 mM HCL and 0.1% non-ionic P 40 in isopropanol). Plates were read on a Biotek HT plate reader at 590 nM with a reference at 620 nM. NE quantitation NE ELISA (BA E-5200) kits were purchased from Rocky Mountain Diagnostics. Plasma was collected at the termination of the study by cardiac puncture using EDTA anticoagulant. Tumour lysates were prepared as described above, but with the addition of 1 mM EDTA and 4 mM Na 2 S 2 O 5 . ELISAs were performed according to manufacturer’s instructions and read with a Biotek HT plate reader. Standard curve analysis was performed on GraphPad software using a four-parameter logistic curve. All readings were normalized to total protein content. Corticosterone quantitation Corticosterone levels were determined from faecal samples collected from mice housed at ST and TT conditions for ~3–4 weeks by ELISA (Cayman). Samples were collected by placing mice in separate clean cages for 15 min. Samples were collected, frozen in dry ice and stored at −80 °C until processing. Corticosterone was extracted by methanol and ELISAs were run as per manufacturer’s instructions. Plates were read at 420 nM and all readings were normalized to faecal mass. Transfection Cells were cultured as described above. MIA PaCa-2 cells were plated into a 96-well plate and allowed to grow until near confluence. Cells were then transfected with pGL4.5 control plasmids (Promega) and Lipofectamine LTX Plus (Invitrogen Life Sciences) in media and selected with 400 μg ml −1 of Hygromycin B. Colonies were isolated and then screened for luminescence activity using D-luciferin (Gold Bio) and read on a Biotek HT plate reader. shADRB2 and scramble constructs were purchased from Origene and transfected into MIA PaCa-2 cells using Fugene HD (Promega); these target sequences are specific for ADRB2 and do not cross-react with ADRB1 or ADRB3. Cells were selected with 2.5 μg ml −1 of puromycin (Stressmarq) and individual GFP-expressing colonies were isolated and screened by flow cytometry as previously described and RT–PCR for knockdown of ADRB2 . RNA was collected using Trizol Reagent (Invitrogen) based on the manufacturer’s protocol. RNA was quantitated by Biotek HT based on A260/A280. About 1 μg of total RNA was used for synthesis of complementary DNA using Superscript III First Strand Synthesis (Invitrogen). PCR products were amplified using Taq polymerase (Invitrogen) and visualized on 2% agarose gel (Invitrogen). Human ADRB2 forward primers: 5′- TTCTTGCTGGCACCCAATGGAAG -3′, Human ADRB2 reverse 5′- CCAGTGAAGTGATGAAGTTGGTG -3′. Mice Female C.B. Igh-1b Icr Tac Prkdc scid mice (6–8 week old) were acquired from Roswell Park Cancer Institute In-house Breeding Services. C57BL/6 mice (6–8 week-old female) were purchased from the National Cancer Institute. All experiments involving mice were performed in accordance with the guidelines established by the Institutional Animal Care and Use Committee at Roswell Park Cancer Institute (Buffalo, NY, USA). Precision Refrigerated Plant-Growth Incubators (Thermo Fisher Scientific) maintained at 22 or 30 °C were modified for additional humidity control using a Top Fin Air Pump AIR 1000 with Top Fin airline tubing. Cages containing experimental mice were housed five to a cage in these incubators under standard light–dark cycles with access to ad libitum water and standard chow (6.2% fat). Subcutaneous tumour models SCID mice were injected s.c. with MIA PaCa-2 (2 × 10 6 cells), BxPC-3 (4 × 10 6 cells) or Pan02 (10 5 cells) suspended in 0.9% sterile saline (Baxter Inc) in the lower left abdomen. Patient xenograft tumours were surgically implanted into the lower right abdomen of SCID mice anesthetized with isofluorane as previously described in ref. 45 . Orthotopic tumour model SCID mice were anesthetized with isofluorane and injected with MIA PaCa-2 luc cells (10 6 ) suspended in reduced growth factor matrigel matrix (BD Biosciences). Mice were given 100 μl of 0.01 mg ml −1 buprenorphine and 100 μl of sterile saline prior to surgery. To access the pancreas, an incision was made on the upper left abdomen and the spleen was gently retracted to expose the pancreas. Tumour cells were injected into the head of the pancreas and the incision was sealed by dissolvable suture (Ethicon) and Vetbond (3 M Animal Care). Tumours were allowed to establish for 2 weeks at which time all mice had detectable tumours and then they were imaged twice weekly with an IVIS-50 system (Perkin Elmer) following injection with 15 mg kg −1 of D -luciferin. Therapeutic studies Mice were implanted with tumours as described above and maintained under standard research facility conditions until tumours had reached ~50 mm 3 . At this point, mice were randomized by tumour volume (calculated by the formula height × height × width/2) and placed into specified temperature controlled incubators. After 3 days, mice were treated with 500 μg of Apo2L/TRAIL daily, 5 mg kg −1 of cisplatin 2–3 times per week, 5 mg ml −1 of nab -paclitaxel every 3 days or saline by i.p. injections. Mice were treated with 100 mg kg −1 erlotinib by gavage and control mice received the vehicle 6% Captisol. In some experiments, 10 mg kg −1 of propranolol or saline was given daily by i.p. in combination with therapies. Tumour growth was monitored by calipers and final tumour mass was measured (Mettler Toledo). For orthotopic studies, mice were placed on a similar treatment schedule and tumour growth was measured weekly by bioluminescence. How to cite this article: Eng, J. W.-L. E. et al . Housing temperature-induced stress drives therapeutic resistance in murine tumour models through β 2 -adrenergic receptor activation. Nat. Commun. 6:6426 doi: 10.1038/ncomms7426 (2015).